Analysis of mitochondrial genome diversity identifies new and ancient maternal lineages in Cambodian aborigines Cambodia harbours a variety of aboriginal (and presumably ancient) populations that have largely been ignored in studies of genetic diversity. Here we investigate the matrilineal gene pool of 1,054 Cambodians from 14 geographic populations. Using mitochondrial whole-genome sequencing, we identify eight new mitochondrial DNA haplogroups, all of which are either newly defined basal haplogroups or basal sub-branches. Most of the new basal haplogroups have very old coalescence ages, ranging from ~55,000 to ~68,000 years, suggesting that present-day Cambodian aborigines still carry ancient genetic polymorphisms in their maternal lineages, and most of the common Cambodian haplogroups probably originated locally before expanding to the surrounding areas during prehistory. Moreover, we observe a relatively close relationship between Cambodians and populations from the Indian subcontinent, supporting the earliest costal route of migration of modern humans from Africa into mainland Southeast Asia by way of the Indian subcontinent some 60,000 years ago. Bordered by Thailand, Laos and Vietnam on the southern coast of the Indochina Peninsula, the Kingdom of Cambodia has a population of about 13.4 million (Cambodia National Census, 2008), 96% of which belongs to Khmer, a result of the historic expansion of the Khmer Empire in the 12th century [1] . Alongside the Khmer, there are 20 minority ethnic groups that reside primarily in the northeastern provinces, colloquially known in Cambodia as aborigines. Linguistically, Austro-Asiatic languages are the most common in Cambodia, being spoken by the Khmer and nearly all the aborigines. Being one of the most ancient language families in eastern Asia, Austro-Asiatic is also spoken in India, Bangladesh and southwestern China, implying that the Austro-Asiatic speaking populations may represent the descendants of the earliest settlers of modern humans who migrated from Africa and entered into eastern Asia about 60,000 years ago (ya) [2] , [3] , [4] . Previous genetic studies of the mitochondrial DNA (mtDNA) and the Y-chromosome diversity of Asian populations suggested that modern humans of ultimate African origin initially entered into the southern part of eastern Asia around 60,000 ya and then migrated northward to mainland East Asia about 40,000 ya [2] , [3] , [5] , [6] , [7] . This southern origin and northward migration were confirmed by a recent analysis of genome-wide sequence variation, in which the Austro-Asiatic speaking populations were found at a basal position in the phylogenetic tree illustrating the genetic relationships among Asian populations. [8] Collectively, currently available genetic data places mainland Southeast Asia (MSEA) and southern China as the potential cradle of modern humans for the initial peopling of eastern Asia. Consequently, revealing the pattern of ancient genetic diversity among early modern human populations is not only informative simply for tracing the prehistoric migrations but also important for understanding the underlying molecular mechanisms of adaptation to the varied environments early human settlers faced along their migratory paths. Though many genetic studies have been conducted in populations from Southeast Asia (for example, populations from Thailand, Laos, Vietnam, Malaysia, Indonesia and other Island of Southeast Asian (ISEA) countries) [9] , [10] , [11] , [12] , [13] , [14] , [15] , [16] , [17] , [18] , there have been only a few studies with limited samples from Cambodia. In previous study, we found a relatively higher genetic diversity among Cambodians (in a relatively small sample comprising 26 male individuals) when compared with the surrounding populations [2] , [3] , [4] , [5] , [19] , an implication of inherited ancient genetic diversity among the Cambodian aborigines. In another study, however, no novel lineages were observed in the scans of mtDNA (31 samples) and Y-chromosome markers (125 samples) [20] , though this was most probably due to a limited sample size and insufficient coverage of aboriginal populations from Cambodia. In this study, to elucidate the genetic background of Cambodian aborigines, we collected a total of 1,054 unrelated samples, representing 13 aboriginal ethnic populations and one Khmer population. These populations are from three provinces in northeastern Cambodia, where nearly 95% of all the aborigines live ( fig. 1 ). We analyse sequence variation within the mtDNA control region (HVS-I and HVS-II) as well as parts of the coding region in all the samples. In addition, we sequence the entire mitochondrial genomes of 98 selected samples. These Cambodian aboriginal mitogenomes reveal four novel basal lineages and a further four novel sub-branches, indicating that present-day Cambodian aborigines still retain ancient genetic polymorphisms in their maternal lineages. 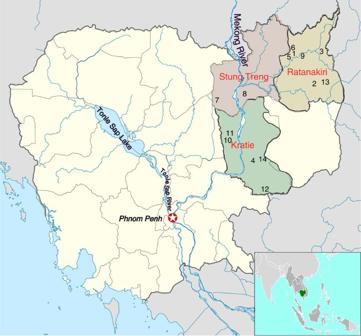Figure 1: Geographic locations of the 14 sampled Cambodian populations. Numbers refer to the populations (1. Brao; 2. Jarai; 3. Kachac; 4. Khmer; 5. Kravet; 6. Kreung; 7. Kuy; 8. Lao; 9. Lun; 10. Mel; 11. Phnong; 12. Stieng; 13. Tompuon; and 14. Kraol). The names of the three northeastern provinces are indicated. Figure 1: Geographic locations of the 14 sampled Cambodian populations. Numbers refer to the populations (1. Brao; 2. Jarai; 3. Kachac; 4. Khmer; 5. Kravet; 6. Kreung; 7. Kuy; 8. Lao; 9. Lun; 10. Mel; 11. Phnong; 12. Stieng; 13. Tompuon; and 14. Kraol). The names of the three northeastern provinces are indicated. Full size image Classification of the Cambodian mtDNA haplogroups Through control region and partial coding region as well as whole-genome sequencing, a total of 1,000 out of 1,054 (94.88%) Cambodian individuals ( Fig. 2 ) were classified into 69 known mtDNA haplogroups/subhaplogroups ( Supplementary Data 1 ), previously identified in Southeast Asian and East Asian populations ( http://www.phylotree.org , mtDNA tree build 15 (30 September 2012)) [21] . The remaining 54 individuals belong to eight novel mtDNA haplogroups newly identified in this study. Overall, the dominant haplogroups observed in the Cambodian populations were B5 (28.08%), F1 (18.22%), M12b (8.25%), R22 (5.79%) and B4 (5.60%), which altogether account for 65.94% (695/1,054) of all samples ( Fig. 2 ). 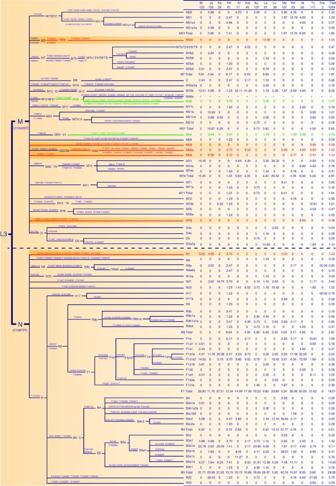Figure 2: Distribution of the mtDNA haplogroups in Cambodian populations. The branches in red colour are the newly defined haplogroups in this study. The branches in green colour are the re-defined haplogroups due to the adding of the Cambodian sequences. The mutations used to define the mtDNA lineages are given along the branches. For transversions, the derived alleles are shown in lowercase. Back-mutations are indicated with a ‘!’ suffix. Population abbreviations: Br, Brao; Ja, Jarai; Ka, Kachac; KH, Khmer; Kr, Kravet; Kre, Kreung; Ku, Kuy; La, Lao; Lu, Lun; Me, Mel; PH, Phnong; St, Stieng; To, Tompuon; and Kra, Kraol. Figure 2: Distribution of the mtDNA haplogroups in Cambodian populations. The branches in red colour are the newly defined haplogroups in this study. The branches in green colour are the re-defined haplogroups due to the adding of the Cambodian sequences. The mutations used to define the mtDNA lineages are given along the branches. For transversions, the derived alleles are shown in lowercase. Back-mutations are indicated with a ‘!’ suffix. Population abbreviations: Br, Brao; Ja, Jarai; Ka, Kachac; KH, Khmer; Kr, Kravet; Kre, Kreung; Ku, Kuy; La, Lao; Lu, Lun; Me, Mel; PH, Phnong; St, Stieng; To, Tompuon; and Kra, Kraol. Full size image We compared the haplogroup profiles between the two non-Austro-Asiatic (Lao and Jarai) and the other Austro-Asiatic populations ( Table 1 ), and no clustering by language families was observed ( Fig. 3 ), implying that there has been extensive genetic exchange among regional populations in Cambodia despite the fact that they belong to different language families. Therefore, these two non-Austro-Asiatic populations were not treated separately in the following analyses. The Kraol population was omitted in the following analyses considering its small size ( n =2). Table 1 The background information of the 14 sampled Cambodian populations. 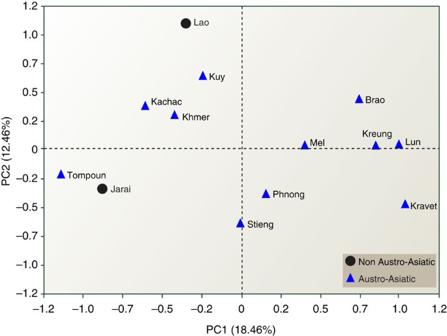Figure 3: Map of principal component analysis among the Cambodian populations. The mtDNA haplogroup frequency data of 13 Cambodian populations is used in the analysis. The Kraol population was excluded due to its small size (n=2). The first and second prinicipal components (PC1 and PC2) explain 18.46 and 12.46% of the genetic variance, respectivley. Full size table Figure 3: Map of principal component analysis among the Cambodian populations. The mtDNA haplogroup frequency data of 13 Cambodian populations is used in the analysis. The Kraol population was excluded due to its small size ( n =2). The first and second prinicipal components (PC1 and PC2) explain 18.46 and 12.46% of the genetic variance, respectivley. Full size image Novel mtDNA basal lineages and sub-branches in Cambodians Using mitochondrial whole-genome sequencing, we identified a total of eight novel lineages that have not been reported or classified previously. Phylogenetic analysis indicated that four of these are novel basal lineages within macrohaplogroup M (designated as M59, M69 and M78) and macrohaplogroup N (designated as N7). Three of the four newly defined lineages (M59, M69 and M78) also included previously reported but unclassified sequences from other Asian populations ( Fig. 4 ). The other four lineages are novel sub-branches of the known M/N haplogroups (designated as M68 (which shares a root with M62), M68a, M3d and M3d1) with all of them also sitting at basal positions within the respective haplogroups. 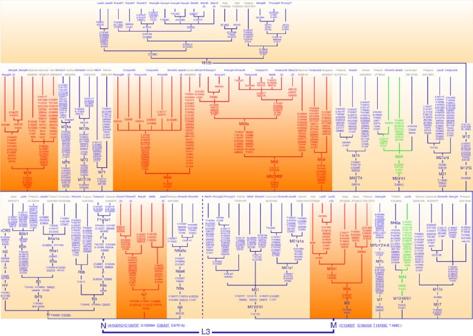Figure 4: Phylogenetic tree based on 133 mitochondrial whole genomes. The tree includes 98 newly sequenced Cambodians genomes and 35 previously reported genomes from other Asian populations (the sample IDs are shown in grey colour). The branches in red colour are the novel basal haplogroups and sub-branches, and the branches in green colour are the re-defined haplogroups due to the adding of the Cambodian sequences. The mutations used to define the mtDNA lineages are given along the branches. For transversions, the derived alleles are shown in lowercase. Back-mutations are indicated with a ‘!’ suffix. Synonymous mutations in the coding region are underlined. The numbers in the brackets are sample size of the haplotypes. Figure 4 illustrates the phylogenetic positions of the eight newly identified haplogroups in Cambodians. Although they only account for a small portion (5.12%) of the Cambodian mtDNA pool, these presumably ancient haplogroups suggest a high genetic diversity due to antiquity of the Cambodian maternal lineages. Figure 4: Phylogenetic tree based on 133 mitochondrial whole genomes. The tree includes 98 newly sequenced Cambodians genomes and 35 previously reported genomes from other Asian populations (the sample IDs are shown in grey colour). The branches in red colour are the novel basal haplogroups and sub-branches, and the branches in green colour are the re-defined haplogroups due to the adding of the Cambodian sequences. The mutations used to define the mtDNA lineages are given along the branches. For transversions, the derived alleles are shown in lowercase. Back-mutations are indicated with a ‘!’ suffix. Synonymous mutations in the coding region are underlined. The numbers in the brackets are sample size of the haplotypes. Full size image Among the four newly identified basal lineages, haplogroup M78 is defined by a mutation motif of A93G-A4164G-A15652G-C16287T–C16327a, which includes three previously unclassified sequences, two from Myanmar (JX289097 and JX289130, NCBI GenBank nucleotide database) and one from Tibet (HM030537) (ref. 22 ), which belong to a M78 sub-branch deeply divergent from the four Cambodian samples of the Stieng ethnic group. The haplogroup M69 is defined by a short mutation motif C4392T-T11365C, which is shared by a sequence (HM596653) from Sumatra (Indonesia) [23] , but with a deep divergence with the twelve sequences from four different Cambodian ethnic groups. The haplogroup M59 is defined by a long motif of A249G-G9380A-T10256C-C11140T-G14040A-T16140C-C16278T, shared by a sequence (JQ702247) from Singapore [24] but with a deep divergence from a Cambodian sample of the Tompoun ethnic group. The haplogroup N7 is a completely new basal lineage within macrohaplogoup N, defined by a long motif of A723G-G6570t-T11617C-A13542G-C14668T-C15945T- G16129A, and, interestingly, it is only observed in Cambodians. A previously identified basal lineage M62 (refs 25 , 26 , 27 ) was joined with the novel lineage M68 (defined by G16255A-T16311C) identified in Cambodians, designated as M62'68, and defined by the mutation motif C150T-T4561C-G7664A. Eleven Lao sequences in Cambodians turned out to belong to a sub-branch of haplogroup M3, designated M3d (defined by T11827C-C16344T), to which also four previously published sequences, JF742206 (Nepal) [28] , FJ770946 (India) [29] , DQ112779 (Brahui, Pakistan) [30] and JF742212 (Nepal) [29] belong. The sequences JF742206 and FJ770946, together with the eleven Cambodian Lao samples, form a M3d sub-branch, designated M3d1 (defined by T10238C-T13820C). In addition, another Cambodian sequence (Lao09) refined the motif of haplogroup M46 (now defined by T146C-C3588T) and showed a deep divergence with a sequence (FJ442939) from Thailand [31] . Two Cambodian sequences (Khmer02 and Jarai06) refined the mutation motif of haplogroup M24 (now defined by T146C-T195C-G5773A-G13359A-T15601C), to which the two previously reported sequences DQ112783 (Cambodia) [30] and JF739543 (Philippines) [32] belong. Collectively, the novel basal mtDNA lineages found in Cambodians suggest that current Cambodian aborigines still carry ancient genetic diversity. Estimated coalescent times of Cambodian mtDNA haplogroups The estimated coalescence ages of the mtDNA haplogroups are listed in Table 2 . Most of the haplogroups are very ancient (>25,000 years), especially the newly identified haplogroups in Cambodians. For example, M78, M69 and M68, three of the newly identified haplogroups, have extremely old coalescence ages (55,188 years, 68,137 years and 82,782 years, respectively), falling into the suggested period of initial peopling of modern humans in eastern Asia [2] , [3] . Two other novel basal lineages in Cambodians are younger but still of considerable age (36,388 years for N7 and 27,594 years for M59). In addition, besides the newly identified mtDNA lineages in Cambodians, the other lineages (previously reported in other Asian populations) also have relatively old coalescence ages, most of them being older than 25,000 years, whereas only two of the observed lineages fell into the Neolithic period (<10,000 years) ( Table 2 ). The old coalescence ages of the mtDNA lineages are consistent with the multiple novel basal lineages found in Cambodians, again suggesting that the Cambodian aborigines are ancient populations. We also used the Bayesian method in BEAST [33] and the maximum likelihood method in PAML [34] for age estimation, and the estimated ages by different methods are consistent ( Table 3 ). Table 2 Estimated time to the most recent common ancestor (TMRCA) of the haplogroups and their haplotype diversity in Cambodians. Full size table Table 3 Comparison of haplogroup ages estimated by three different methods. Full size table Phylogeographic patterns of the dominant haplogroups To delve into the phylogeographic and migratory patterns of the major haplogroups in Cambodians, we constructed networks ( Fig. 5 ) and frequency contour maps ( Fig. 6 ) of the haplogroups by combining all available data in Asian populations. B5a was the most dominant haplogroup (28.08%) in Cambodians ( Fig. 2 and Table 2 ) and was also prevalent in southern China (Yunnan, Guangxi, Guangdong and Hainan provinces), northern Laos and southern Vietnam, but rare in northern Asian populations ( Supplementary Data 2 ). The reduced median network of haplogroup B5a ( Fig. 5a ) indicates that the core haplotype of B5a is mostly shared among the southern populations in eastern Asia, suggesting a southern origin of this mtDNA lineage. The contour map of B5a indicates that the origin of B5a probably lies in MSEA (probably Cambodia), as reflected by the diversified haplotypes ( Fig. 5a ) and the high level of haplotype diversity (0.8364) of the haplogroup B5a HVS-I sequences in Cambodians ( Table 2 ), which is comparable to the diversity levels of B5a in Vietnam (0.8824) and Thailand (0.8444). The estimated coalescence age of B5a in Cambodians is 34,220 years, which is much older than its coalescence age in other populations (for example, 16,200 years in ISEA [11] and 26,000 years in Japan [31] ), and close to the proposed time of the initial northward migration of modern humans in eastern Asia [2] , [3] , [5] . In addition, the star-like network of B5a suggests a relatively recent expansion of this lineage. 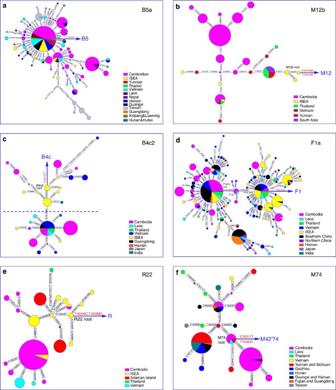Figure 5: Haplotype networks of the major haplogroups in Cambodians and other Asian populations. The HVS-I sequences are used to construct the networks of B5a (a), M12b (b), B4c2 (c), F1a (d), R22 (e) and M74 (f). Different colours represent different geographic populations. Figure 5: Haplotype networks of the major haplogroups in Cambodians and other Asian populations. The HVS-I sequences are used to construct the networks of B5a ( a ), M12b ( b ), B4c2 ( c ), F1a ( d ), R22 ( e ) and M74 ( f ). Different colours represent different geographic populations. 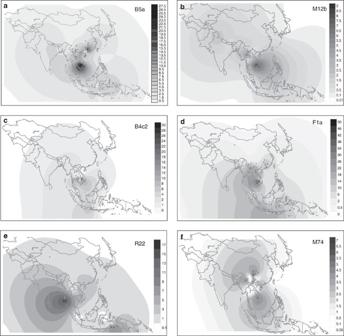Figure 6: Contour maps of the major haplogroups in Cambodians and other Asian populations. The haplotype frequencies are used to construct the contour maps of B5a (a), M12b (b), B4c2 (c), F1a (d), R22 (e) and M74 (f). The black dots indicate the geographic locations of the analysed populations. The bars indicate the haplotype frequency spectrum. Full size image Figure 6: Contour maps of the major haplogroups in Cambodians and other Asian populations. The haplotype frequencies are used to construct the contour maps of B5a ( a ), M12b ( b ), B4c2 ( c ), F1a ( d ), R22 ( e ) and M74 ( f ). The black dots indicate the geographic locations of the analysed populations. The bars indicate the haplotype frequency spectrum. Full size image F1 is another prevalent haplogroup in Cambodians (18.22%), of which the most common sub-haplogroup is F1a ( Fig. 2 ). The reduced median network of F1a showed that there are two major clusters (F1a* and F1a1a) ( Fig. 5d ), both of which have star-like shapes, suggesting recent expansions, consistent with the pattern seen in B5a ( Fig. 5a ). A previous study reported that the sister branches of F1a, that is, F1b and F1c, are largely restricted to southern China, and F1 and F1a were suggested to have a possible origin in this region [11] . Also, due to the high diversity of root types in Indochina, F1a1a was suggested to have expanded from MSEA to ISEA during the Holocene [11] . F1a1a is a prevalent haplogroup in Southeast Asia; besides Cambodia, it is also common in Thailand and in aboriginal Senoi groups of the Malay Peninsula [12] , and the coalescence age of F1a1a was estimated to be 9,000 years in ISEA [11] . F1a (including F1a1a) has a peak frequency (48%) in the Stieng ethnic group of Cambodia. Both F1a* and F1a1a in Cambodians have ancient coalescence ages (around 60,000 and 48,000 years, respectively) ( Table 2 ), which are much older than their ages in other MSEA regions. Hence, F1a probably originated in MSEA (with Cambodia as a candidate region) and expanded to ISEA, which is also reflected by the F1a contour map ( Fig. 6d ). M12b is a Cambodian-specific haplogroup with moderate prevalence (8.25%) in Cambodians, which was firstly defined by Fucharoen et al . [35] , with sporadic presence in northern India [25] , southwestern China (Yunnan province) [36] , [37] , [38] , northern Thailand [35] , [39] , Laos [9] and ISEA [12] , [40] . The reduced median network of M12b ( Fig. 5b ) suggests that the M12b haplotypes in ISEA (mainly Indonesia) were derived from those in Cambodians, and an eastward migration can be inferred from the contour map of M12b ( Fig. 6b ). In addition, the phylogenetic structure of M12b derived from sequencing the mitogenomes of 19 representative Cambodian samples clearly supports a Cambodian origin of this mtDNA lineage ( Fig. 4 ). Haplogroup B4c2, which was first defined by Tanaka et al . [31] , accounts for 5.03% in Cambodians. It is also prevalent (10.12%) in southern Vietnam and Thailand [14] and widely distributed in southern China and other Southeast Asian countries [20] ( Fig. 5c ). The reduced median network of B4c2 indicated that the haplotypes from ISEA are sitting at the root position of the network, and there are two distinctive subclusters separated by a transversion (C16184a) ( Fig. 5c ), which seems to suggest an ISEA origin of this haplogroup. However, the reported coalescence age of B4c2 in ISEA is around 21,000 years [11] , which is much younger than the B4c2 age in Cambodians (~45,000 years) ( Table 2 ), thus favouring an MSEA origin. The haplogroup R22 accounts for 5.79% in Cambodians, which is a relatively young lineage (~19,000 years in Cambodians) ( Table 2 ). The reduced median network of R22 ( Fig. 4e ) suggests an ISEA origin of this lineage with the root haplotypes mostly observed in ISEA and the Andaman Islands, consistent with a previous dating of ~29,000 years in ISEA [11] . The contour map of R22 indicates a westward migration from ISEA to MSEA ( Fig. 6e ). The haplogroup M74 (4.93%) represents another lineage showing a migration from other regions to Cambodia. It was first reported by Kong et al . [22] based on mitochondrial whole-genome sequencing, and was suggested to have a southern China origin, dated to 43,000 years ago. The reduced median network of M74 ( Fig. 5f ) agrees with this view with most of the core haplotypes being distributed in southern China. The contour map of M74 ( Fig. 6f ) suggests two possible expansion centres, one in southern China and another one in Cambodia. The coalescence time of M74 in Cambodians was estimated at ~39,000 years, younger than that in southern China ( Table 2 ). Hence, a southern China origin of this haplogroup seems more congruent with the currently available data from Asian populations. There are also other minor haplogroups in Cambodians (R9b, N9a and M71) showing an into-Cambodia migratory pattern [12] , [14] , [17] . Genetic relationship of Cambodians with nearby populations Finally, to examine the genetic relationship of Cambodians with surrounding populations, we conducted a principal component analysis (PCA) based on the mtDNA haplogroup frequencies of Cambodians and 225 different Asian populations, and the result is shown in Fig. 7 . The first component (PC1), which explains 18.40% of the genetic variance, separates the northern and southern Asian populations. The second component (PC2, 10.86%) indicates divergence among the southern populations. Intriguingly, the Cambodian populations are clustered with populations from India (Dravidian, Indo-European and Austro-Asiatic speaking populations), Andaman Islands (one Austro-Asiatic speaking population), Australia (aborigines) and Madagascar, but relatively diverged from the other southern populations (Austronesian, Daic and Hmong-Mien speaking populations in MSEA and southern China). In addition, within the Austro-Asiatic language family, Cambodians are closer to the Austro-Asiatic speaking populations from India and the Andaman Islands than to those from MSEA and southern China. 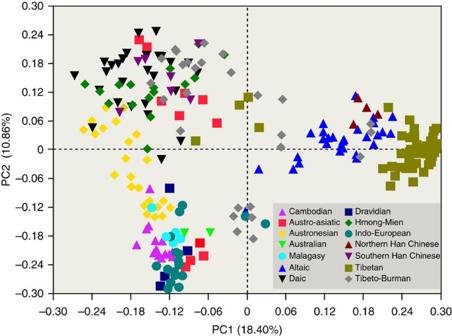Figure 7: Map of the principal component analysis among Cambodians and 225 other Asian populations. Non-Cambodian populations were grouped by language families. The four Austro-Asiatic populations (red squares) located in the lower left corner are from India (three populations) and the Andaman Islands (one population). The first and the second components explain 18.40 and 10.86% of the genetic variance, respectively. Figure 7: Map of the principal component analysis among Cambodians and 225 other Asian populations. Non-Cambodian populations were grouped by language families. The four Austro-Asiatic populations (red squares) located in the lower left corner are from India (three populations) and the Andaman Islands (one population). The first and the second components explain 18.40 and 10.86% of the genetic variance, respectively. Full size image Inference of demographic changes To infer demographic changes through time for Cambodian aborigines, we carried out Bayesian skyline plot (BSP) [41] using all Cambodian mtDNA HVS-I sequences ( Fig. 8 ). The BSP showed a relatively constant female effective population size in the past 50,000 years, suggesting that the Neolithic agricultural diffusion had a minor impact on the Cambodian aborigines. 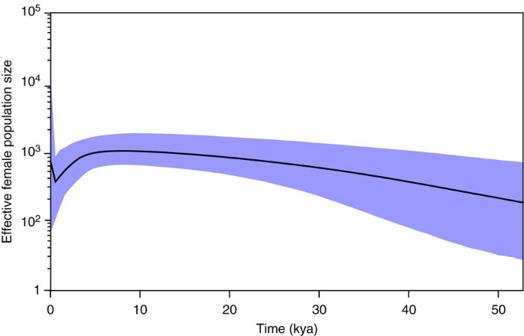Figure 8: Bayesian skyline plot of changes of female effective population size through time for Cambodian aborigines. The plot was generated using 1,054 Cambodian HVS-I (16,038–16,462) sequences. The MCMC chain was run for 1 × 108steps, with sampling of parameters every 2,500 steps, and the initial 1 × 107steps were discarded as burn-in. The purple area reflects the s.d. values of the estimated effective populations sizes. Figure 8: Bayesian skyline plot of changes of female effective population size through time for Cambodian aborigines. The plot was generated using 1,054 Cambodian HVS-I (16,038–16,462) sequences. The MCMC chain was run for 1 × 10 8 steps, with sampling of parameters every 2,500 steps, and the initial 1 × 10 7 steps were discarded as burn-in. The purple area reflects the s.d. values of the estimated effective populations sizes. Full size image Through an extensive sampling in Cambodian aborigines and high-resolution mtDNA diversity analyses, we showed that Cambodian aboriginal populations still carry ancient sequence polymorphisms in their maternal lineages, suggesting that Cambodia was probably located in the region where the earliest modern human settlers initially populated eastern Asia. We identified eight novel mtDNA lineages in Cambodians, including four basal haplogroups and four sub-branches. This was rather unexpected given the extensive surveys of mtDNA diversity that have already been conducted in many MSEA regions (Thailand, Vietnam, Myanmar and Laos) and southern China [6] , [7] , [9] , [11] , [14] , [22] , [35] , [36] , [37] , [38] , [42] , [43] , [44] , [45] . The dating of the mtDNA haplogroups supports the antiquity of Cambodian populations, with most of the estimated haplogroup ages exceeding 25,000 years. In particular, the ages of the newly defined basal haplogroups M59, M69, M78 and N7 were estimated between ~36,000 and ~68,000 years ago ( Table 2 ), falling within the suggested time period of the earliest settlement of modern humans in eastern Asia [3] , [4] . Notably, although most of the newly defined basal haplogroups in Cambodians also exist in other Asian populations, the Cambodian sequences are highly diverged from the non-Cambodian sequences for M59, M69 and M78 ( Fig. 4 ), therefore, it is unlikely that these ancient mtDNA lineages were brought into Cambodia only recently via migration. Until now, no ancient human fossils or cultural relics beyond the Neolithic time have yet been discovered in Cambodia [46] , [47] , probably due to the limited excavations conducted by archaeologists and/or the tropical environments in Cambodia, which are not ideal for fossil and relic preservation. Besides the newly identified mtDNA lineages, many dominant haplogroups in Cambodia, which are shared with populations in MSEA and southern China, probably also originated locally in Cambodia. As reflected by the contour maps of the major haplogroups ( Fig. 6 ), most of the dominant haplogroups in Cambodians (B5a, F1a, M12b and B4c2) have high frequencies and high haplotype diversities in Cambodia as compared with the surrounding regions, an implication of a Cambodian dispersal centre of these haplogroups, northward to mainland East Asia and southward to ISEA. Notably, there are also less-prevalent haplogroups, which seem to have been brought into Cambodia from other regions, including R22, M74 and several other minor haplogoups (R9b, N9a and M71). The genetic relationships inferred from the PCA map among extended Asian populations are consistent with the proposed antiquity of the Cambodian aborigines. In the PCA map ( Fig. 7 ), Cambodians are clustered with populations from the Indian subcontinent, the Andaman Islands, Australia (aborigines) and Madagascar, congruent with the widely accepted costal migratory route of modern humans, which starting in Africa advanced through the Indian subcontinent and into MSEA around 60,000 years ago [3] , [48] . This clustering pattern tends to support a single early migration wave of modern humans from Africa to eastern Asia [8] , [48] though a recent analysis of the genome of an aboriginal Australian suggested multiple dispersals [49] . In addition, the findings of ancient maternal lineages in Cambodians supports the idea of a MSEA dispersal centre of modern humans in eastern Asia, consistent with the proposed southern origin and early northward migrations of modern humans in mainland East Asia inferred from Y-chromosome data [2] . Hence, further studies of the aboriginal populations from other Southeast Asian countries, such as Myanmar, may reveal more unidentified ancient mtDNA lineages. Alternatively, Cambodia also experienced recent influence from India. Cambodia historically had a highly Indianized state known as Funan (first to sixth century) and its successor Chenla (late sixth to the early ninth century), harbouring a culture similar to that in India. Substantial Indian immigration during the first to thirteenth century was suggested to have made a hefty contribution to the modern gene pool of Cambodians [50] . However, as we argued above, most of the dominant haplogoups in Cambodians showed an out-of-Cambodia expansion pattern, and the influence of the suggested relatively recent gene flows from India does not seem to have had a large impact on the Cambodian aborigines, at least regarding their matrilineal ancestry. In conclusion, Cambodia harbours ancient and indigenous mtDNA haplogroups, which have accumulated abundant mutations that show patterns of long-term in situ evolution. Many of the prevalent mtDNA haplogroups in ISEA and mainland East Asia probably originated in MSEA (presumably Cambodia). Hence, the Cambodian aborigines are important ethnic populations for reconstructing the genetic makeup of early modern human settlers in Asia. Sample collection We collected 5 ml of blood samples from a total of 1,054 unrelated individuals (693 females and 361 males) from Cambodia. These samples were from 14 geographic populations, including 13 aboriginal populations and 1 Khmer population from three provinces in northeastern Cambodia ( Fig. 1 ). Written informed consents were obtained from all sampled Cambodian individuals, and the study protocol was approved by the Internal Review Board of Kunming Institute of Zoology, Chinese Academy of Sciences. As shown in Table 1 , except for Jarai and Lao, which belong to Austronesian and Daic language families, respectively, all the other 12 populations belong to the Mon-Khmer branch of the Austro-Asiatic family. MtDNA sequencing and genotyping Following the previously described method [45] , for all the 1,054 samples, we first sequenced the mtDNA HVS-I (range: 16,038–16,462) and HVS-II (range: 65–417) regions, as well as a coding region (range: 10,220–10,610) containing two sites, 10,398 and 10,400, diagnostic for the macrohaplogroups N and M, respectively. We next sequenced several diagnostic-site-containing coding regions to define the mtDNA haplogroup of each individual ( Supplementary Data 1 ). Based on this strategy, 860 individuals could be assigned to a known mtDNA haplogroup. From the remaining 194 samples of unknown haplogroups, we selected 75 representative samples, together with 4 samples of known haplogroups, which were subjected to whole-mitochondrial genome sequencing. Based on the phylogenetic information gained from the newly sequenced mtDNA genomes, we next sequenced at least one specific coding-region position in the remaining 119 samples to define their haplogroups ( Supplementary Data 1 ). Moreover, to clarify the phylogeny of haplogroup M12b, which is specific to Cambodians, we additionally conducted whole-genome sequencing of 19 samples belonging to this haplogroup. In total, we acquired the mitochondrial whole-genome sequences of 98 Cambodian individuals. The protocol for mitochondrial whole-genome sequencing was adopted from a published study [51] involving amplification of two overlapping fragments each of 8.5 kb in length. For the newly discovered mtDNA haplogroups, the nomenclature follows the system suggested by van Oven [26] . We also collected previously published mtDNA data from extensive array of Asian populations (21,100 samples from 225 populations), mostly containing HVS and partial coding-region sequences ( Supplementary Data 2 ). Phylogenetic analysis and haplogroup age estimation To determine the phylogenetic positions of the newly discovered Cambodian haplogroups, we employed 133 complete mtDNA genome sequences (including the 98 newly sequenced mitogenomes in the present study and the 35 previously reported mitogenomes from Asia [14] , [17] , [22] , [23] , [24] , [25] , [28] , [29] , [30] , [32] , [42] , [43] , [48] , [52] ) to construct the phylogenetic tree. From the NCBI nucleotide database ( http://www.ncbi.nlm.nih.gov ), we selected 35 mitogenomes, including 10 reported but unclassified mitogenomes related with the newly defined haplogroups in Cambodians. We also randomly selected 25 reported mitogenomes that share known haplogroups with Cambodians. With these 35 reference mitogenomes, the phylogenetic positions of the Cambodian sequences can be indicated ( Fig. 4 ). To reveal the detailed structure of the major haplogroups among Cambodians, based on the HVS-I sequence data, reduced median networks were constructed using the programme NETWORK version 4.6.1.0 (Fluxus Engineering) [53] . The unbiased HVS-I haplotype diversity was calculated with DnaSP (verion 5.10) [54] following the method described by Nei [55] . The coalescence time to the most recent common ancestor of each haplogroup was estimated using the ρ ± σ statistics. We also used the Bayesian method and the maximum likelihood method embedded in BEAST [33] and PAML [34] , respectively, for age estimation. The mutation rates of 16,677 years, 7,884 years and 3,624 years per mutation were used for HVS-I (16,051–16,400), coding region (577–16,023) synonymous mutations and entire mtDNA genome, respectively [56] . For Bayesian and maximum likelihood, the haplogroups with whole mtDNA genome data and a sample size of n >5 were analysed, and the estimated ages are consistent with those by the rho method ( Table 3 ). To establish the genetic relationships between Cambodians and other Asian populations, we performed PCA based on the frequencies of mtDNA haplogroups according to the method developed by Richards et al . [57] in the MVSP3.13 software. Contour maps of the major haplogroups in Cambodians were constructed using Golden Software Surfer 10.0 (Golden Software Inc., USA) with the Kriging algorithm. Bayesian skyline plot To reconstruct the demographic changes through time for Cambodian aborigines, we reconstructed BSP [41] in BEAST (version 1.7.5) [33] with MCMC algorithms [58] . The BSP was generated using 1,054 Cambodian HVS-I (16038–16462) sequences. A strict molecular clock with a fixed rate of 1.784 × 10 −7 substitutions per site per year [56] was applied. The MCMC chain was run for 1 × 10 8 steps, with sampling of parameters every 2,500 steps, and the initial 1 × 10 7 steps were discarded as burn-in. In all runs, the effective sample size for eight parameters of interest was over 200. The BSP was visualized with Tracer 1.5 ( http://tree.bio.ed.ac.uk/ software/tracer), and the female effective population size was plotted on a log scale by assuming a female generation time of 25 years. Population growth rate was calculated from the skyline plot using method described elsewhere [59] . Accession Numbers : Sequence data for the 98 mtDNA whole-genome sequences and the 1,054 HVS-I sequences have been deposited in GenBank/EMBL/DDBJ nucleotide core database under accession numbers KC505067 to KC505122 , KC887456 to KC887497 and KC504013 to KC505066 . How to cite this article: Zhang, X. et al. Analysis of mitochondrial genome diversity identifies new and ancient maternal lineages in Cambodian aborigine. Nat. Commun. 4:2599 doi: 10.1038/ncomms3599 (2013).